The phosphatase Dullard negatively regulates BMP signalling and is essential for nephron maintenance after birth Most kidney nephron components, including glomeruli and renal tubules, derive from the metanephric mesenchyme. The overall differentiation into each component finishes at birth, but the molecular events linking the perinatal and adult kidneys remain elusive. Dullard was cloned from Xenopus kidneys, and encodes a phosphatase that negatively regulates BMP signalling. Here we report that Dullard deletion in the murine metanephric mesenchyme leads to failure of nephron maintenance after birth, resulting in lethality before adulthood. The nephron components are lost by massive apoptosis within 3 weeks after birth, leading to formation of a large hollow with a thin-layered cortex and medulla. Phosphorylated Smad1/5/8 is upregulated in the mutant nephrons, probably through cell-autonomous inhibitory effects of Dullard on BMP signalling. Importantly, administration of the BMP receptor kinase inhibitor LDN-193189 partially rescued the defects caused by Dullard deletion. Thus, Dullard keeps BMP signalling at an appropriate level, which is required for nephron maintenance in the postnatal period. A mammalian kidney contains approximately one million nephrons, which are functional units consisting of glomeruli, proximal tubules, loop of Henle, distal tubules and collecting ducts. During development, the nephron structure is formed by reciprocally inductive interactions between two precursor tissues, the metanephric mesenchyme and the ureteric bud [1] . The former contains multipotent nephron progenitors that express several transcription factors including Six2 and Sall1 [2] , [3] . A lineage tracing study demonstrated that the Six2-expressing mesenchyme gives rise to most parts of the nephron epithelia, including glomerular podocytes, parietal cells of Bowman’s capsule and tubular cell lineages (proximal tubules, loop of Henle and distal tubules), but not the collecting duct cells [2] . The collecting duct epithelia are derived from the ureteric bud that expresses Hoxb7 (ref. 4 ). These nephron-forming processes start at around weeks 4–5 of gestation and finish at around weeks 34–36 of gestation in humans [5] , compared with embryonic day (E) 10.5 and within a few days after birth, respectively, in mice [6] . Therefore, many factors that have impacts on kidney development and the nephron number during this time window have been identified [7] . After this period, the nephron progenitors disappear and no more new nephrons are formed, but the kidney continues to grow until adulthood. However, it remains largely unclear how postnatal nephrons are maintained and develop to the adult kidney. We consistently use Xenopus embryos to isolate new genes involved in kidney development, which has led to the identification of Sall1 , deletion of which causes kidney agenesis [8] . Dullard , which contains a C-terminal phosphatase-like domain, was also isolated from Xenopus embryos and is expressed in the kidney of tadpoles [9] . Dullard promotes ubiquitin-mediated proteasomal degradation of BMP type II receptor and dephosphorylates BMP type I receptor, thereby preventing BMP signalling [10] . This is consistent with the observation that Dullard knockdown in Xenopus embryos inhibits neural development in vivo , which requires inhibition of BMP activity [10] . A recent study also showed that Dullard is required for negative regulation of BMP signalling during wing vein formation in Drosophila [11] . However, the function of Dullard in mammals, including that in the kidney, has remained unknown for more than 10 years since the gene was cloned. Several BMP ligands and their receptors and antagonists are expressed in the developing mouse kidney. For example, BMP7 is expressed in both the metanephric mesenchyme and ureteric bud, and the phenotypes of Bmp7 -deficient mice suggest that BMP7 is essential for maintaining the nephrogenic progenitors during kidney development [12] , [13] , [14] . BMP4 inhibits ectopic formation of ureteric buds [15] and deletion of GREMLIN1, a BMP4 antagonist expressed in the metanephric mesenchyme, leads to impaired outgrowth of the ureteric bud and renal agenesis [16] . Given the importance of BMP signalling in mammalian kidney development and the involvement of Dullard in BMP signalling, we generated mutant mice lacking Dullard in the kidney. In contrast to our expectations, metanephric mesenchyme-specific deletion of Dullard did not show any kidney defects until birth. However, the mutant mice exhibited severe nephron loss within several weeks after birth through enhanced BMP signalling, thereby providing a molecular link between the perinatal and adult kidneys. Mice lacking Dullard in their nephrons die before adulthood We examined Dullard expression during kidney development by utilizing Dullard-lacZ mice, in which β-galactosidase gene was inserted into the Dullard locus. X-gal staining at E17.5 showed ubiquitous signals in all areas of the kidney, including the metanephric mesenchyme ( Fig. 1a , arrowhead) and ureteric buds ( Fig. 1a , arrow). At postnatal day (P) 14, the signals were still detected in all areas, including the cortex, outer medulla and inner medulla ( Fig. 1b ). Ubiquitous expression of Dullard in the embryonic and postnatal kidneys was confirmed by in situ hybridization ( Supplementary Fig. S1a ). 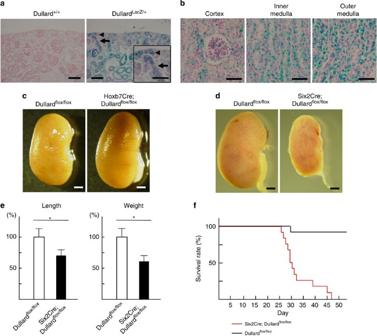Figure 1: Mice lackingDullardin their nephrons die before adulthood. (a) X-gal staining of E17.5 kidneys from wild-type (Dullard+/+) andDullardlacZ/+heterozygous mice. Arrows: metanephric mesenchyme; arrowheads: ureteric bud. Scale bar, 100 μm. Inset: high-magnification image of the nephrogenic zone. Scale bar, 50 μm. (b) X-gal staining of a 2-week-oldDullardlacZ/+heterozygous kidney showinglacZexpression in all renal tubule segments throughout the cortex, outer medulla and inner medulla. Scale bar, 100 μm. (c) Macroscopic evaluation of 28-day-oldDullardflox/floxandHoxb7Cre;Dullardflox/floxmutant kidneys. No obvious abnormalities are observed. Scale bar, 1 mm. (d) Macroscopic views ofDullardflox/floxandSix2Cre;Dullardflox/floxkidneys at birth and at 28 days of age, showing a significant size reduction of the mutant kidney at P28. Scale bar, 1 mm. (e) Measurements of the renal length and weight at P28 show obvious size reductions of theSix2Cre;Dullardflox/floxmutant kidneys (n=6 in each group). Mean±s.d., *P<0.001. (f) A Kaplan–Meier survival analysis shows a significant difference between control (n=18) andSix2Cre;Dullardflox/floxmutant mice (n=12) (two-sided log-rank test,P<0.001). The median survival time ofSix2Cre;Dullardflox/floxmutant mice is 33.3 days. Figure 1: Mice lacking Dullard in their nephrons die before adulthood. ( a ) X-gal staining of E17.5 kidneys from wild-type ( Dullard +/+ ) and Dullard lacZ/+ heterozygous mice. Arrows: metanephric mesenchyme; arrowheads: ureteric bud. Scale bar, 100 μm. Inset: high-magnification image of the nephrogenic zone. Scale bar, 50 μm. ( b ) X-gal staining of a 2-week-old Dullard lacZ/+ heterozygous kidney showing lacZ expression in all renal tubule segments throughout the cortex, outer medulla and inner medulla. Scale bar, 100 μm. ( c ) Macroscopic evaluation of 28-day-old Dullard flox/flox and Hoxb7Cre ; Dullard flox/flox mutant kidneys. No obvious abnormalities are observed. Scale bar, 1 mm. ( d ) Macroscopic views of Dullard flox/flox and Six2 Cre; Dullard flox/flox kidneys at birth and at 28 days of age, showing a significant size reduction of the mutant kidney at P28. Scale bar, 1 mm. ( e ) Measurements of the renal length and weight at P28 show obvious size reductions of the Six2Cre ; Dullard flox/flox mutant kidneys ( n =6 in each group). Mean±s.d., * P <0.001. ( f ) A Kaplan–Meier survival analysis shows a significant difference between control ( n =18) and Six2Cre ; Dullard flox/flox mutant mice ( n =12) (two-sided log-rank test, P <0.001). The median survival time of Six2Cre ; Dullard flox/flox mutant mice is 33.3 days. Full size image Germline deletion of Dullard exhibited lethality at the post-implantation stage (RN, unpublished data). To gain insights into the roles of Dullard during kidney development, we generated two types of conditional mutant mice. A floxed allele of Dullard was generated ( Supplementary Fig. S1b–d ) and first crossed with Hoxb7Cre mice expressing Cre recombinase in the ureteric bud-derived lineage [17] . However, Hoxb7Cre; Dullard flox/flox mice were obtained at a Mendelian frequency when examined at 8 weeks after birth ( Dullard flox/+ , 8/36 (22.2%); Dullard flox/flox , 8/36 (22.2%); Hoxb7Cre; Dullard flox/+ , 11/36 (30.6%); Hoxb7Cre; Dullard flox/flox , 9/36 (25%)). The mice showed no apparent abnormalities in the kidneys ( Fig. 1c and Supplementary Fig. S2a ) with normal cortical and medullary structures ( Supplementary Fig. S2b ), and survived for over 1 year, although successful deletion of Dullard was confirmed by genomic PCR ( Supplementary Fig. S2c ). Thus, Dullard is dispensable for the ureteric bud-derived lineage, including the collecting ducts. Next, we crossed the floxed allele of Dullard with Six2Cre mice expressing Cre recombinase in the nephron progenitors in the metanephric mesenchyme [2] ( Supplementary Fig. S2d ). The Six2Cre; Dullard flox/flox mice showed similar-sized kidneys to control mice at P0 ( Fig. 2a , upper panel), and survived until weaning at 3 weeks after birth. However, the mutant kidney size was significantly reduced at P28 ( Fig. 1d , left panel) and the kidney weight was nearly half of the control kidney weight ( Fig. 1e , right panel). The mutant mice started to die after weaning, and all the mutant mice had died before 8 weeks of age with a median survival of 33.3 days ( Fig. 1f , n =12). 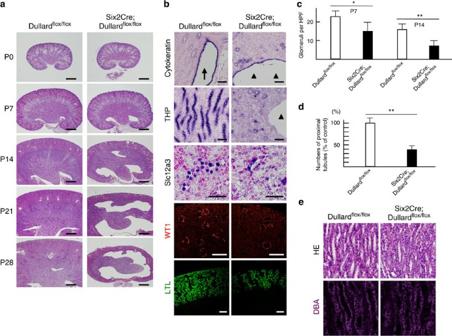Figure 2: Loss of nephron components inDullardmutant mice. (a) Haematoxylin and eosin (HE) staining of control and mutant kidneys at different time points after birth. All images were taken at the same magnification. Scale bar, 100 μm. TheSix2Cre;Dullardflox/floxmutant kidneys become smaller than the control kidneys over time. Note that a cavity appears at P14 and expands thereafter. (b) The cells lining the cavity (arrowheads), as well as the pelvic epithelia (arrow), are positive for cytokeratin. Immunostaining for Tamm–Horsfall protein (THP) (thick ascending limb of the loop of Henle), WT1 (glomerular podocytes) and LTL (proximal tubules) andin situhybridization ofSlc12a3(distal tubules) show a reduction in mesenchyme-derived nephron lineages in the mutant kidneys at P14. Scale bar, 100 μm. (c) The numbers of glomeruli are significantly reduced in the mutant kidneys at P7 and P14 (n=4 in each group). Mean±s.d., *P<0.05. **P<0.001. (d) The numbers of LTL-positive proximal tubules at P21 were counted. Relative numbers was calculated by setting the numbers inDullardflox/floxmice at 100% (n=4 in each group). Mean±s.d., **P<0.001. (e) HE and DBA staining shows that the collecting ducts are not impaired in the mutant kidneys. Scale bars, 50 μm. Figure 2: Loss of nephron components in Dullard mutant mice. ( a ) Haematoxylin and eosin (HE) staining of control and mutant kidneys at different time points after birth. All images were taken at the same magnification. Scale bar, 100 μm. The Six2Cre ; Dullard flox/flox mutant kidneys become smaller than the control kidneys over time. Note that a cavity appears at P14 and expands thereafter. ( b ) The cells lining the cavity (arrowheads), as well as the pelvic epithelia (arrow), are positive for cytokeratin. Immunostaining for Tamm–Horsfall protein (THP) (thick ascending limb of the loop of Henle), WT1 (glomerular podocytes) and LTL (proximal tubules) and in situ hybridization of Slc12a3 (distal tubules) show a reduction in mesenchyme-derived nephron lineages in the mutant kidneys at P14. Scale bar, 100 μm. ( c ) The numbers of glomeruli are significantly reduced in the mutant kidneys at P7 and P14 ( n =4 in each group). Mean±s.d., * P <0.05. ** P <0.001. ( d ) The numbers of LTL-positive proximal tubules at P21 were counted. Relative numbers was calculated by setting the numbers in Dullard flox/flox mice at 100% ( n =4 in each group). Mean±s.d., ** P <0.001. ( e ) HE and DBA staining shows that the collecting ducts are not impaired in the mutant kidneys. Scale bars, 50 μm. Full size image Nephron components are lost in Dullard mutant mice Although the Six2Cre; Dullard flox/flox kidneys were almost indistinguishable from the control kidneys up to P7, a cavity appeared in the outer medulla at P14 ( Fig. 2a ). This cavity was connected, in both the lateral and corticomedullary axes, to the enlarged pelvic space ( Supplementary Fig. S3a ), and the cells lining the cavity were positive for cytokeratin, a marker for pelvic epithelia ( Fig. 2b ). The cavity expanded, and eventually resulted in a large hollow with a thin-layered cortex and an overall reduced kidney size at P28 ( Fig. 2a ). At P14, the formation of the Tamm–Horsfall protein-positive thick ascending limb of the loop of Henle was significantly impaired in the outer medullary region adjacent to the cavity ( Fig. 2b ). Furthermore, we found that the other nephron components were also reduced in the Dullard mutant mice at this stage. The numbers of glomeruli in the mutant kidneys were 48% of the numbers in the control kidneys at P14 ( Fig. 2b ). The numbers of Lotus tetragonolobus lectin (LTL)-positive proximal tubules ( Fig. 2b ) and Slc12a3 -positive distal tubules ( Fig. 2b ) were also reduced. Thus, it is likely that gradual loss of nephron components precedes the cavity formation. Indeed, we were able to detect reduced numbers of glomeruli as early as P7 ( Fig. 2c ). In contrast, Dolichos biflorus agglutinin (DBA)-positive collecting ducts were relatively unaffected even at P21 ( Fig. 2e ), which was consistent with the mesenchyme-specific deletion of Dullard . Dilatation of the ureters in the Dullard mutants was undetectable, despite the enlarged cavity in the kidneys at P21 ( Supplementary Fig. S3b ). Staining with an anti-smooth muscle actin antibody showed that the development of the ureteral wall was also unaffected. Thus, the phenotypes of the Dullard mutants were unlikely to be caused by obstruction or malformation of the lower urinary tracts. These findings suggest that the severe cavity formation in the Dullard mutant kidneys could be secondarily caused by progressive loss of nephron components, including glomeruli, proximal and distal tubules, and the loop of Henle located in the cortex and outer medullary regions. Apoptotic cell death in Dullard mutant nephrons To determine whether the observed phenotype was caused by decreased proliferation of nephrons, sections of control and mutant kidneys were stained for Ki-67 and phosphorylated histone H3 (PHH3). However, we did not detect any significant differences between the two groups in either the cortex or outer medulla ( Fig. 3a ). By contrast, significant numbers of cleaved caspase-3-positive cells were detectable throughout the cortex and outer medulla in the mutant kidneys, while only a few positive cells were detectable in the control kidneys ( Fig. 3c ), suggesting that apoptotic cell death occurred in the Dullard mutant kidneys. To determine the identity of these apoptotic cells, we introduced a yellow fluorescent protein (YFP) lineage reporter [18] into the Dullard mutant mice. In the Six2Cre; R26RYFP mice, all the cells derived from the Six2-positive metanephric mesenchyme were labelled with YFP, and a few cleaved caspase-3-positive cells were detected in YFP-positive mesenchyme-derived nephrons ( Supplementary Fig. S3c ). In contrast, cleaved caspase-3-positive cells were detected in S ix2Cre; Dullard flox/flox ; R26RYFP mice as early as P7, and all the signals overlapped with YFP ( Fig. 3d ), suggesting that mesenchyme-derived nephrons lacking Dullard passed into apoptotic cell death in a cell-autonomous manner. As expected, cleaved caspase-3-positive cells were almost undetectable in the DBA-positive collecting ducts in both the control and mutant kidneys ( Fig. 3d ). Infiltration of macrophages and formation of blood vessels were not enhanced in the regions adjacent to the cavity ( Supplementary Fig. S3d,e ). Considering the marked apoptosis in the nephron lineage and the absence of lower urinary tract obstruction, it is likely that the parenchymal shrinkage initially occurs through nephron loss, followed by secondary enlargement of the pelvic cavity. 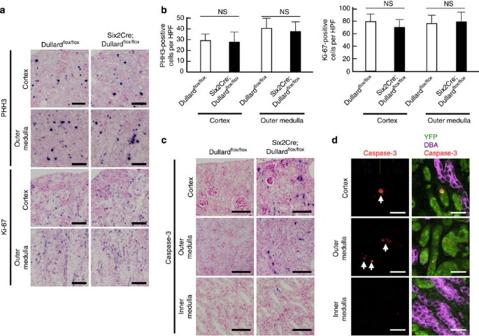Figure 3: Apoptotic cell death occurs inDullardmutant nephrons. (a) Immunostaining for PHH3 and Ki-67 in the 14-day-old cortex and outer medulla. Scale bar, 100 μm. (b) The numbers of PHH3- or Ki-67-positive proliferating cells do not differ between the control and mutant kidneys (n=3 in each group). Mean±s.d., NS, not significant. (c) Cleaved caspase-3-positive apoptotic cells are increased in the 14-day-old mutant cortex and outer medulla, but not in the inner medulla. Scale bar, 100 μm. (d) Cleaved caspase-3-positive cells overlap with YFP-positive mesenchyme-derived cells (green), but not with DBA-positive ureteric bud-derived cells (purple), in 7-day-oldSix2Cre; Dullardflox/flox; R26RYFPmutant kidneys. Scale bar, 100 μm. Figure 3: Apoptotic cell death occurs in Dullard mutant nephrons. ( a ) Immunostaining for PHH3 and Ki-67 in the 14-day-old cortex and outer medulla. Scale bar, 100 μm. ( b ) The numbers of PHH3- or Ki-67-positive proliferating cells do not differ between the control and mutant kidneys ( n =3 in each group). Mean±s.d., NS, not significant. ( c ) Cleaved caspase-3-positive apoptotic cells are increased in the 14-day-old mutant cortex and outer medulla, but not in the inner medulla. Scale bar, 100 μm. ( d ) Cleaved caspase-3-positive cells overlap with YFP-positive mesenchyme-derived cells (green), but not with DBA-positive ureteric bud-derived cells (purple), in 7-day-old Six2Cre; Dullard flox/flox ; R26RYFP mutant kidneys. Scale bar, 100 μm. Full size image BMP signalling is enhanced in Dullard mutant nephrons Studies in Xenopus and Drosophila have suggested that Dullard is a negative regulator of BMP signalling [10] , [11] . First, we examined the messenger RNA (mRNA) expression levels of BMP2 , BMP4 and BMP7 in the kidneys from P0 to P21. The levels of BMP2 and BMP7 were highest at P0 and decreased during the first 3 weeks after birth ( Supplementary Fig. S4a ). By contrast, BMP4 mRNA remained relatively constant during this period ( Supplementary Fig. S4a ). The expression levels of these ligand mRNAs were comparable between the control and Dullard mutant kidneys ( Supplementary Fig. S4b ). Next, we examined phosphorylated Smad1/5/8 (p-Smad1/5/8), which indicates canonical BMP signalling. In the Dullard mutant kidneys at P7, we observed an increase in p-Smad1/5/8 specifically in the epithelial tubules located in the cortex and outer medulla ( Fig. 4a ). By contrast, p-Smad1/5/8 was expressed at similar levels in the medulla, where collecting ducts are enriched, of the control and mutant kidneys. These observations were confirmed by western blot analysis of whole kidney lysates, which demonstrated marked increases in p-Smad1/5/8 in the Dullard mutant kidneys at P7 and P0 ( Fig. 4b and Supplementary Fig. S5a ). We further examined this effect in the presence of the YFP indicator, and confirmed that most of the increased p-Smad1/5/8 signals overlapped with YFP, indicating that mesenchyme-derived nephrons showed enhanced BMP signalling ( Fig. 4c ). Therefore, mesenchyme-derived nephrons lacking Dullard exhibited increased BMP signalling and apoptotic cell death, which could lead to the nephron loss and cavity formation. The increased p-Smad1/5/8 staining was not observed at E17.5, which is consistent with the postnatal onset of the phenotype. Although BMP signalling is also mediated by mitogen-activated protein kinases (MAPK) pathways, including p38 MAPK, there was no difference in the levels of phosphorylated p38 MAPK (p-p38 MAPK) between the control and mutant kidneys ( Fig. 4b ). 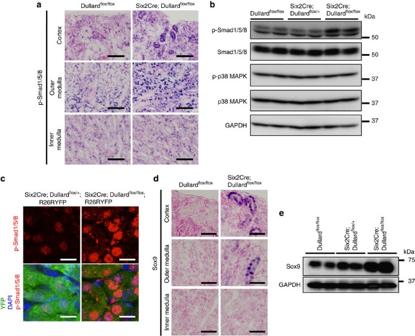Figure 4: Enhanced BMP signalling inDullardmutant nephrons. (a) Immunostaining for p-Smad1/5/8 (blue) shows increased signals in the cortex and outer medulla, but not in the inner medulla, of theDullardmutant kidneys. Nuclei were counterstained with nuclear fast red. Scale bar, 100 μm. (b) Western blot analysis of p-Smad1/5/8, Smad1/5/8, p-p38 MAPK, and p38 MAPK in kidney extracts from 7-day-old mice. Note the increase in p-Smad1/5/8 in the mutant mice. The data represent typical results from two mice of each genotype in three independent experiments. GAPDH was evaluated as a loading control. (c) p-Smad1/5/8-positive cells (red) overlap with YFP-positive mesenchyme-derived cells (green) in 7-day-oldSix2Cre; Dullardflox/flox; R26RYFPmutant kidneys. Scale bar, 10 μm. (d) Immunostaining for Sox9 shows increased signals in the cortex and outer medulla, but not in the inner medulla, of the 7-day-old mutant kidney. Scale bar, 50 μm. (e) Western blot analysis of Sox9 using kidney extracts of 7-day-old mice. Note the Sox9 increase in the mutant mice. The data represent typical results for two mice of each genotype from three independent experiments. GAPDH, glyceraldehyde 3-phosphate dehydrogenase. Figure 4: Enhanced BMP signalling in Dullard mutant nephrons. ( a ) Immunostaining for p-Smad1/5/8 (blue) shows increased signals in the cortex and outer medulla, but not in the inner medulla, of the Dullard mutant kidneys. Nuclei were counterstained with nuclear fast red. Scale bar, 100 μm. ( b ) Western blot analysis of p-Smad1/5/8, Smad1/5/8, p-p38 MAPK, and p38 MAPK in kidney extracts from 7-day-old mice. Note the increase in p-Smad1/5/8 in the mutant mice. The data represent typical results from two mice of each genotype in three independent experiments. GAPDH was evaluated as a loading control. ( c ) p-Smad1/5/8-positive cells (red) overlap with YFP-positive mesenchyme-derived cells (green) in 7-day-old Six2Cre; Dullard flox/flox ; R26RYFP mutant kidneys. Scale bar, 10 μm. ( d ) Immunostaining for Sox9 shows increased signals in the cortex and outer medulla, but not in the inner medulla, of the 7-day-old mutant kidney. Scale bar, 50 μm. ( e ) Western blot analysis of Sox9 using kidney extracts of 7-day-old mice. Note the Sox9 increase in the mutant mice. The data represent typical results for two mice of each genotype from three independent experiments. GAPDH, glyceraldehyde 3-phosphate dehydrogenase. Full size image We further investigated the downstream genes affected by the lack of Dullard in the postnatal kidney. We examined the BMP signalling targets known in other biological settings [19] , [20] . While Id1 and Id2 remained unchanged in the mutant kidneys, Sox9 was significantly upregulated in the mutant kidneys at P7 ( Supplementary Fig. S4c ). Immunostaining revealed Sox9 expression in the cortex and outer medulla in the Dullard mutant kidneys, in the same regions where the increased p-Smad1/5/8 was detected, whereas no expression was observed in the control kidneys ( Fig. 4d ). The kinetics of the Sox9 increase in the mutant kidneys was delayed compared with that of the p-Smad1/5/8 activation. While the p-Smad1/5/8 increase was already detected at P0, there was no increase in Sox9 at P0 ( Supplementary Fig. S5b,c ), and it was only expressed in the ureteric bud tips in both the control and mutant kidneys ( Supplementary Fig. S5d ). These findings suggest that Sox9 could reflect the enhanced BMP signalling in the mutant kidneys, although it is unlikely to be a direct downstream target of the BMP signalling. Cell-autonomous inhibition of BMP signalling by Dullard To examine whether Dullard directly regulates the BMP signalling, we overexpressed Flag-tagged Dullard in the BMP-responsive mouse cell line C3H10T1/2 and generated multiple clones ( Fig. 5a ). Addition of BMP4 caused an increase in p-Smad1/5/8 after 30 min of incubation in the control clones. However, this increase was markedly inhibited in the clones overexpressing Dullard ( Fig. 5b ). When the cells were cultured for 3 days in the presence of BMP4, a Sox9 increase was observed in the control clones ( Fig. 5c ), as previously reported [20] , [21] . Dullard overexpression also inhibited this increase, consistent with the Sox9 upregulation in the Dullard mutant kidneys. These findings suggest that Sox9 could be one of the genes activated at the later phase of BMP signal transduction. 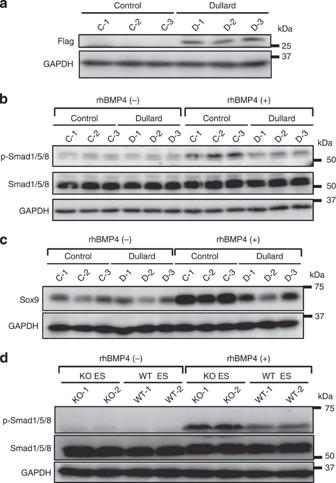Figure 5: Dullard-mediated inhibition of BMP signalling is cell-autonomous. (a) Western blot analysis of three independent C3H10T1/2 clones transfected with the empty vector (C-1, C-2 and C-3) or the vector containing Flag-tagged Dullard (D-1, D-2 and D-3). (b) Dullard overexpression inhibits BMP-dependent phosphorylation of Smad1/5/8 in C3H10T1/2 cells. Each clone was treated with rhBMP4 (50 ng ml−1) for 30 min, and the lysate was immunoblotted with antibodies for the indicated proteins. (c) Dullard overexpression inhibits Sox9 upregulation in C3H10T1/2 cells after 3 days of incubation with BMP4 (50 ng ml−1). (d) Two each of wild-type andDullard-null ES clones were treated with rhBMP4 (50 ng ml−1) for 30 min, and their lysates were immunoblotted with antibodies for the indicated proteins. Note the enhanced p-Smad1/5/8 in theDullard-null ES cells. Figure 5: Dullard-mediated inhibition of BMP signalling is cell-autonomous. ( a ) Western blot analysis of three independent C3H10T1/2 clones transfected with the empty vector (C-1, C-2 and C-3) or the vector containing Flag-tagged Dullard (D-1, D-2 and D-3). ( b ) Dullard overexpression inhibits BMP-dependent phosphorylation of Smad1/5/8 in C3H10T1/2 cells. Each clone was treated with rhBMP4 (50 ng ml −1 ) for 30 min, and the lysate was immunoblotted with antibodies for the indicated proteins. ( c ) Dullard overexpression inhibits Sox9 upregulation in C3H10T1/2 cells after 3 days of incubation with BMP4 (50 ng ml −1 ). ( d ) Two each of wild-type and Dullard -null ES clones were treated with rhBMP4 (50 ng ml −1 ) for 30 min, and their lysates were immunoblotted with antibodies for the indicated proteins. Note the enhanced p-Smad1/5/8 in the Dullard -null ES cells. Full size image We further performed a loss-of-function experiment using embryonic stem (ES) cells. Cre recombinase was introduced using an adenovirus into ES cells derived from Dullard flox/flox blastocysts, and the resultant Dullard -null ES cells were obtained at a high frequency (46 of 48 colonies). The morphology and growth rate of these Dullard mutant clones were not apparently different from those of the Dullard flox/flox clones. When the Dullard -null ES cells were treated with BMP4 for 30 min, the increase in p-Smad1/5/8 was enhanced compared with the control clones ( Fig. 5d ). These findings suggest that Dullard inhibits BMP signalling in a cell-autonomous manner. BMP inhibition rescues kidney defects in Dullard mutant mice To examine whether enhanced BMP signalling is a major cause of the nephron loss in the Dullard mutant mice, we performed daily injections (from P1 to P20) of LDN-193189, a selective inhibitor of BMP type I receptor kinases [22] , into mothers nursing pups, including Six2Cre; Dullard flox/flox mutant mice. This treatment had no detectable adverse effects on the control mice, but resulted in suppression of the enhanced BMP signalling ( Supplementary Fig. S6a ) and a partial rescue of the kidney defects in the Dullard mutant mice ( Fig. 6 ). Histologically, the cavity in the outer medulla was much smaller and the cortex thinning was less prominent at P21, compared with untreated mutant mice ( Fig. 6a ). Staining of proximal tubules enriched in the cortex confirmed the recovery of the cortex thickness ( Fig. 6b ), and the numbers of proximal tubules were significantly rescued in the treated mutant mice ( Fig. 6c ). Other nephron components, such as the loop of Henle and distal tubules, were also modestly restored ( Fig. 6d ). The partial rescue of the phenotype by LDN-193189 administration may reflect incomplete inhibition of the BMP activity under our experimental conditions. Nonetheless, our findings indicate that the enhanced BMP signalling in the absence of Dullard does indeed cause the nephron loss. 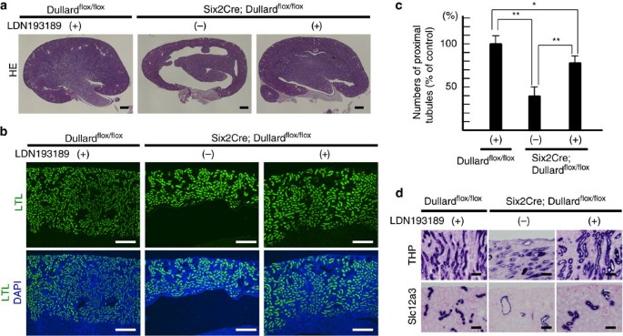Figure 6: BMP signalling inhibition rescues kidney defects inDullardmutant mice. (a) Haematoxylin and eosin (HE) staining of kidneys at P21 from control and mutant mice with or without LDN-193189 treatment for 3 weeks after birth. The treated mutant kidneys show a much smaller cavity in the outer medulla. One representative image for a mouse of each genotype is shown. Scale bar, 500 μm. (b) LTL staining (green) at P21 shows restored thickness of the cortex, which is rich in proximal tubules. Scale bar, 100 μm. (c) The numbers of LTL-positive proximal tubules at P21 are partially restored in the treated mutant kidneys compared with the untreated mutant kidneys (n=4 in each group). Mean±s.d., *P<0.05, **P<0.001. (d) The impairments of the thick ascending limb of the loop of Henle (Tamm–Horsfall protein (THP)-positive) and distal tubules (Slc12a3-positive) are partially restored by the treatment at P21. Scale bar, 100 μm. HE, Haematoxylin and eosin. Figure 6: BMP signalling inhibition rescues kidney defects in Dullard mutant mice. ( a ) Haematoxylin and eosin (HE) staining of kidneys at P21 from control and mutant mice with or without LDN-193189 treatment for 3 weeks after birth. The treated mutant kidneys show a much smaller cavity in the outer medulla. One representative image for a mouse of each genotype is shown. Scale bar, 500 μm. ( b ) LTL staining (green) at P21 shows restored thickness of the cortex, which is rich in proximal tubules. Scale bar, 100 μm. ( c ) The numbers of LTL-positive proximal tubules at P21 are partially restored in the treated mutant kidneys compared with the untreated mutant kidneys ( n =4 in each group). Mean±s.d., * P <0.05, ** P <0.001. ( d ) The impairments of the thick ascending limb of the loop of Henle (Tamm–Horsfall protein (THP)-positive) and distal tubules (Slc12a3-positive) are partially restored by the treatment at P21. Scale bar, 100 μm. HE, Haematoxylin and eosin. Full size image Inhibitory activity of Dullard against BMP signalling was reported in Xenopus and Drosophila [10] , [11] . Our in vivo and in vitro data indicate that this function of Dullard is conserved in mammals. We found that deletion of Dullard in the metanephric mesenchyme-derived tissues resulted in severe apoptosis and nephron loss within several weeks after birth. BMP activity was enhanced in the mutant nephron epithelia and a BMP signal inhibitor partially rescued the phenotype, suggesting that proper control of BMP signalling is essential for nephron maintenance in the neonatal kidney. The late onset of the phenotype was unexpected, considering the importance of BMP activity during embryonic kidney development. Proper levels of BMP4 and BMP7 are required for kidney formation, and deletion of BMP modulators, such as Gremlin and Crossveinless , results in kidney agenesis or hypoplasia at birth [16] , [23] . By contrast, the Dullard mutant mice exhibited no obvious defects until birth, but started to lose their nephrons at 2 weeks after birth, which is different from all phenotypes in mice lacking other BMP-related molecules. It is possible that other BMP modulators could compensate for the Dullard deletion until birth, but not after birth. Alternatively, Dullard could fine-tune the BMP signalling in specialized biological settings instead of being a general BMP signalling inhibitor. Although our data for C3H10T1/2 and ES cells suggest the former possibility, the relationship between Dullard and BMP signalling in vivo remains to be elucidated. Nevertheless, it is interesting that BMP signalling should be suppressed to an appropriate level for postnatal nephron maintenance. Since Bmp2 and Bmp7 decreased after birth, while Bmp4 remained constant, in both the control and mutant mice, the enhancement of BMP signalling in the Dullard mutant mice could arise through decreased degradation of BMP receptors, as proposed previously [10] . Although we did not detect significant increases in the BMP receptor levels in the Dullard mutant kidneys at P7 ( Supplementary Fig. S6b ), it is still possible that slightly increased amounts of the receptors, which were undetectable by western blot analyses, could lead to the increased BMP signalling, because of the high turnover rate of the receptors. Alternatively, Dullard could negatively regulate BMP signalling though Lipin, a phosphatidate phosphatase [24] , [25] . Dullard is involved in the regulation of nuclear membrane biogenesis by dephosphorylating Lipin in cultured cells [24] . It was also reported that Drosophila dullard functions via lipin to regulate the production of diacylglycerol from phosphatidic acid and maintains the proper lipid composition of the nuclear membrane at nuclear pore complexes [25] . Thus, impairment of this process could affect the nuclear translocation of phosphorylated Smad proteins [11] . BMP is associated with apoptotic cell death in many biological processes [26] , such as in the web of the developing fingers [27] , and thus the enhanced BMP activity is likely to induce apoptosis in the mutant kidneys. It remains to be clarified why the neonatal nephron epithelia are sensitive to BMP signalling and undergo the apoptotic process. All components of the nephron showed activation of Smad1/5/8 and caspase-3, while ureteric bud-specific deletion of Dullard exhibited no apparent phenotypes, although a sensitivity difference could also exist among the nephron epithelia, considering that the cavity always started to form in the outer medulla. Regulated BMP signal activation temporally and spatially in vivo would help to solve this question. Congenital abnormalities of the renal–urinary tract system occur in 1 of 500 newborns [28] . Nephronophthisis (NPHP) in humans is a major paediatric kidney disease that shows nephron loss prominently in the outer medullary region, kidney size reduction and renal failure predisposing the patients to hypertension [29] . To date, 12 different genes (NPHP1–12) have been identified with mutations in patients with NPHP [30] . Although many of the identified genes are considered to be associated with ciliopathies, the causative genes are still unknown in ~70% of patients with NPHP or NPHP-like diseases [31] . Mutations in Dullard , as well as enhanced BMP activity, should be searched for in patients who are diagnosed with NPHP or NPHP-like diseases. In summary, Dullard controls BMP signalling at an appropriate level, which is required for proper maintenance of nephrons at the postnatal period. Further studies will lead to elucidation of the molecular differences between embryonic and postnatal kidney development. It would also be interesting to delete Dullard at the adult stage to elucidate the molecular differences between neonatal and adult kidneys, as it is well established that BMP is protective against renal injuries or diseases [32] , [33] , [34] . In addition, the floxed allele of Dullard could be used to examine a variety of biological settings that involve BMP signalling. Generation of Dullard floxed mice The generation of conventional Dullard mutant mice, including Dullard-lacZ , will be described elsewhere. The Dullard-flox targeting vector was constructed by incorporating the 5′ and 3′ homology arms into a vector containing a loxP-loxP-frt-Neo-pA-frt-pA cassette and pMC1DTA ( Supplementary Fig. S1a ). The loxP sequences were placed so that exons 2, -3 and -4 were excised by Cre-mediated recombination to disrupt the C-terminal phosphatase-like domain domain. Seven ES cell clones were correctly targeted ( flox/+ ) and confirmed by Southern blot analysis ( Supplementary Fig. S1b ). The Dullard flox/+ ES cells were injected into 8-cell-stage embryos to generate chimeric mice. The chimeras were crossed with C57BL/6 mice to obtain Dullard floxed heterozygous offspring ( Dullard flox/+ mice; Acc. No. CDB0564K: http://www.cdb.riken.jp/arg/mutant%20mice%20list.html ). The offspring were genotyped by genomic PCR ( Supplementary Fig. S1c ) using primer sets for the wild-type allele (F1 and R1) or Dullard floxed allele (F1 and R2). The primer sequences used for PCR were as follows: F1, 5′-CTGCAGGTGGTAATAGACAAACAC-3′; R1, 5-CTGTTCATTTAGAGAACCCCAACTA-3′; and R2, 5′-CTGTCCATCTGCACGAGACT-3′. The PCR products were 210 bp for the wild-type allele and 573 bp for the Dullard floxed allele. For detecting Cre-mediated deletion of the Dullard genome, the following primers were used: F2, 5′-CCGCACGTCTAAGAAACCAT-3′; and R2 (509 bp). Six2Cre and R26RYFP mice were provided by Dr Andrew McMahon (Harvard Medical School) and Dr Frank Costantini (Columbia University), respectively [2] , [18] . Hoxb7Cre mouse was obtained from the Jackson Laboratory [17] . X-gal staining Kidneys from Dullard-lacZ mice were embedded in optimal cutting temperature (OCT) compound (Tissue Tek) and cryosectioned at 20-μm thickness. For X-gal staining, the sections were fixed in 2% formaldehyde/0.4% glutaraldehyde in PBS for 5 min, washed three times with PBS, and stained with 5 mM K3Fe[CN]6, 6.5 mM K4Fe[CN]6, 6.2 mM MgCl 2 , and 0.1% X-gal (1 mg ml −1 ) for 2 h at 37 °C. In situ hybridization and immunohistochemistry Samples were fixed in 10% formalin and processed for paraffin-embedded sectioning. In situ hybridization and immunostaining were performed using an automated Discovery System (Roche) according to the manufacturer’s protocols [35] , [36] . The Slc12a3 probe was isolated by PCR. For fluorescence immunohistochemistry, paraffin-embedded sections were deparaffinized and autoclaved at 121 °C for 5 min in citrate buffer (pH 6.0). After incubation in blocking solution for 1 h at room temperature, the sections were incubated overnight with primary antibodies at 4 °C, followed by incubation with secondary antibodies conjugated with Alexa Fluor 488 or 594 (Life Technologies). The lectins and primary antibodies used were: LTL (Vector Laboratories; 1:300); DBA (Vector Laboratories; 1:500); anti-THP (Biomedical Technologies; 1:200); anti-WT1 (Santa Cruz Biotechnology; 1:100); anti-Slc12a3 (Millipore; 1:500); anti-Ki-67 (Vector Laboratories; 1:100); anti-PHH3 (Millipore; 1:100); anti-GFP (Abcam; chicken-derived; 1:500); anti-cleaved caspase-3 (Cell Signalling Technology; 1:300); anti-p-Smad1/5/8 (Cell Signalling Technology; 1:100); anti-Sox9 (Millipore; 1:300) and anti-CD31 (Abcam; 1:100). Frozen sections were used for staining with an anti-F4/80 antibody (Serotec; 1:100). Counting of stained cells in sections Ki-67-positive cells and PHH3-positive cells were counted in three randomly selected cortical and outer medullary fields from each mouse. The numbers of glomeruli were determined by counting the WT1-stained glomeruli in four randomly selected cortical fields from each mouse. The numbers of proximal tubules were determined by a modification of a previously described method [8] . Briefly, LTL staining was performed in the midline sections, and the LTL-stained proximal tubules were counted in three randomly selected cortical fields from each kidney. Quantitative reverse transcription–PCR Total RNA was isolated from frozen kidneys (one kidney sample per mouse) using the TRIzol reagent (Life Technologies) according to the manufacturer’s instructions. The RNA concentration was determined by ultraviolet spectrophotometry, and the RNA integrity was analysed by agarose gel electrophoresis. Quantitative reverse transcription–PCR (qRT–PCR) was performed as previously described [35] . The primers used are shown in Supplementary Table S1 . All samples were normalized by the β-actin expression using the relative standard curve method. We carried out three independent experiments, and representative data are shown. Sorting of kidney cells The E18.5 kidney was dissociated into single cells by collagenase type XI (Sigma) and trypsin treatment. For the ureteric bud-derived lineage, the samples were stained with biotinylated DBA (Vector) and phycoerythrin-conjugated streptavidin, and sorted using a FACSAria (Becton Dickinson), followed by qRT–PCR of Dullard . For sorting of the metanephric mesenchyme, the GFP in Six2Cre mice was used, as the GFP-Cre fusion was driven by the Six2 promoter [2] . Expression of Six2 and Wnt11 was examined to prove the successful sorting of the mesenchyme and the ureteric bud, respectively. Western blotting Kidneys were snap-frozen in liquid nitrogen and stored at −80 °C until analysis. For each mouse, one frozen kidney was dissociated on ice using a sonicator (amplitude of 40 for 10 × 5 s) in lysis buffer (50 mM Tris–HCl pH 7.5, 100 mM NaCl, 5 mM EDTA, 0.5% Triton X-100, 10% glycerol, 1% protease inhibitor cocktail (Sigma) and 1% phosphatase inhibitor cocktail (Pierce)). The protein concentrations were determined using a Protein Assay Kit (Bio-Rad) according to the manufacturer’s protocol. SDS-sample buffer was added to the samples and boiled for 5 min. The western blotting analyses were carried out using a standard protocol. The primary antibodies used were as follows: anti-p-Smad1/5/8 (Cell Signalling Technology; 1:1,000); anti-Smad1/5/8 (Santa Cruz Biotechnology; 1:1,000); anti-p-p38 MAPK (Cell Signalling Technology; 1:1,000); anti-p38 MAPK (Cell Signalling Technology; 1:1,000); anti-Sox9 (Millipore; 1:1,000); anti-GAPDH (Ambion; mouse-derived; 1:10,000); anti-BMPRIA (Abcam; 1:200); anti-BMPR2 (Cell Signalling Technology; 1:500); and anti-Flag (Sigma; mouse-derived; 1:10,000). Signals were detected using an enhanced chemiluminescence (ECL) plus western blotting detection system (GE Healthcare) and exposure to an LAS-3000 system (Fuji Film). Cell culture and transfection Mouse fibroblast C3H10T1/2 cells were maintained in DMEM supplemented with 10% foetal bovine serum at 37 °C in a 5% CO 2 atmosphere. Flag-tagged Dullard was cloned into the pCAG-ires puro vector [36] , [37] . Cells were transfected with the empty vector or the vector containing Flag-tagged Dullard using Lipofectamine 2000 (Life Technologies) and selected in the presence of puromycin. Multiple independent clones were isolated. The cells were cultured in the absence or presence of 50 ng ml −1 BMP-4 (R&D Systems) and harvested with lysis buffer as described above. Establishment of Dullard flox/flox and Dullard -null ES cells Dullard flox/flox ES cells were established by modification of a previously described protocol [38] , [39] . Blastocysts obtained from intercrosses of Dullard floxed homozygous mice were cultured in DMEM containing β-mercaptoethanol, non-essential amino acids, pyruvate, 14% Knockout Serum Replacement (Life Technologies), 1% serum, 1 × 10 3 U ml −1 LIF, 5 μM CHIR99021, and 3 μM PD0325901 for 10 days in a gelatine-coated 48-well plate. The ES cells were then suspended using 0.125% trypsin/EDTA and expanded. The resultant ES cells were infected with an adenovirus expressing Cre recombinase as previously described [40] to obtain Dullard -null ES cells. LDN-193189 treatment of new-born mice A selective inhibitor of BMP type I receptor kinases, LDN-193189 (Wako), was dissolved in sterile endotoxin-free H 2 O at a concentration of 0.55 mg ml −1 and the pH was adjusted to 6.8. Lactating females were administered a daily intraperitoneal injection of LDN-193189 (2.5 mg kg −1 body weight). At day 21, the mice were euthanized, and their kidneys were dissected and subjected to histochemistry as described above. Two treated Dullard flox/flox mice, three untreated Dullard mutant mice, and two treated mutant mice were examined. Statistical analyses We measured the statistical significance of compared measurements with the Student’s two-tailed t -test. How to cite this article: Sakaguchi, M. et al . The phosphatase Dullard negatively regulates BMP signalling and is essential for nephron maintenance after birth. Nat. Commun. 4:1398 doi: 10.1038/ncomms2408 (2013).